Inhibition of vemurafenib-resistant melanoma by interference with pre-mRNA splicing Mutations in the serine/threonine kinase BRAF are found in more than 60% of melanomas. The most prevalent melanoma mutation is BRAF(V600E), which constitutively activates downstream MAPK signalling. Vemurafenib is a potent RAF kinase inhibitor with remarkable clinical activity in BRAF(V600E)-positive melanoma tumours. However, patients rapidly develop resistance to vemurafenib treatment. One resistance mechanism is the emergence of BRAF alternative splicing isoforms leading to elimination of the RAS-binding domain. Here we identify interference with pre-mRNA splicing as a mechanism to combat vemurafenib resistance. We find that small-molecule pre-mRNA splicing modulators reduce BRAF3–9 production and limit in-vitro cell growth of vemurafenib-resistant cells. In xenograft models, interference with pre-mRNA splicing prevents tumour formation and slows growth of vemurafenib-resistant tumours. Our results identify an intronic mutation as the molecular basis for a RNA splicing-mediated RAF inhibitor resistance mechanism and we identify pre-mRNA splicing interference as a potential therapeutic strategy for drug resistance in BRAF melanoma. The serine/threonine kinase BRAF is a proto-oncogene that acts in the MAP kinase pathway, connecting mitogen signals to transcriptional regulatory networks of cell proliferation. Mutations in BRAF are highly prevalent and are found in more than 60% of melanomas [1] , [2] , [3] . The most common melanoma mutation is BRAF(V600E), which constitutively activates downstream MAPK signalling [4] . Vemurafenib is a potent short-term therapeutic agent for treatment of BRAF(V600E)-positive melanoma [5] . However, patients invariably develop resistance to the drug [6] , [7] , [8] , [9] , [10] , [11] , [12] , [13] , [14] , [15] . Resistance may arise by re-activation of mitogen-activated protein (MAP)/extracellular signal-regulated kinases (ERK) signalling pathways [7] , [11] , including upstream rat sarcoma (RAS) activation by RAS mutation, upregulation of Receptor Tyrosine Kinases [6] , [14] , amplification of BRAF(V600E) [12] , activating mutations in MAPK/ERK kinase (MEK) [8] and epidermal growth factor receptor (EGFR) [15] , [16] . In ∼ 30% of resistant tumours, resistance to the RAF inhibitor vemurafenib is conferred by alternative splicing via generation of BRAF isoforms lacking the RAS-binding domain (RBD) encoded by exons 3–5 (refs 17 , 18 , 19 ; Fig. 1a ). In the absence of the RBD, these BRAF isoforms dimerize even in the presence of low levels of RAS and confer drug resistance [13] . 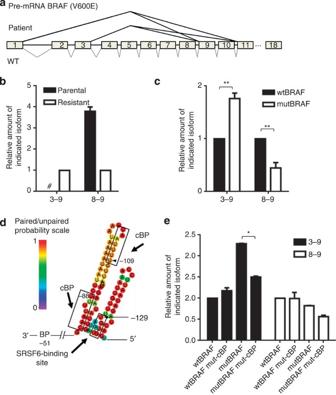Figure 1: A branch-point mutation in the resistant C3 cell line promotes BRAF3–9 splicing. (a) Schematic representation of AS events detected in vemurafenib-resistant melanoma patients. Only introns are drawn to scale, intron 1=63 kbp. (b) Quantitative qPCR analysis of parental and resistant C3 cells. Indicated values represent isoform values normalized to total BRAF mRNA. Isoform levels in resistance C3 cell line was set to 1, #Signal below detection limit. (c) U2OS cells were transfected with wt or mutant BRAF reporter. mRNA levels were assessed after 48 h using qPCR, indicated values represent isoform values normalized to the total amount of green fluorescent protein (GFP) mRNA. Isoform levels in wtBRAF were set to 1. (d) Secondary structure of the 3′ SS of intron 8. Colour-coded pairing probability of individual nucleotides is indicated. (e) U2OS cells were transfected with the indicated BRAF reporter. mRNA levels were assessed after 48 h using qPCR, BRAF3–9 isoform values are normalized to the total amount of GFP mRNA. Isoform levels in wtBRAF were set to 1. (b,cande) Values represent the means of three independent experiments ±s.d. (*P<0.05, **P<0.01,t-test). Figure 1: A branch-point mutation in the resistant C3 cell line promotes BRAF3–9 splicing. ( a ) Schematic representation of AS events detected in vemurafenib-resistant melanoma patients. Only introns are drawn to scale, intron 1=63 kbp. ( b ) Quantitative qPCR analysis of parental and resistant C3 cells. Indicated values represent isoform values normalized to total BRAF mRNA. Isoform levels in resistance C3 cell line was set to 1, #Signal below detection limit. ( c ) U2OS cells were transfected with wt or mutant BRAF reporter. mRNA levels were assessed after 48 h using qPCR, indicated values represent isoform values normalized to the total amount of green fluorescent protein (GFP) mRNA. Isoform levels in wtBRAF were set to 1. ( d ) Secondary structure of the 3′ SS of intron 8. Colour-coded pairing probability of individual nucleotides is indicated. ( e ) U2OS cells were transfected with the indicated BRAF reporter. mRNA levels were assessed after 48 h using qPCR, BRAF3–9 isoform values are normalized to the total amount of GFP mRNA. Isoform levels in wtBRAF were set to 1. ( b , c and e ) Values represent the means of three independent experiments ±s.d. (* P <0.05, ** P <0.01, t -test). Full size image Here we have explored the use of splicing modulation as a means to overcome vemurafenib resistance. We show that a point mutation in intron 8 of the BRAF gene mediates the resistance to vemurafenib in a drug-resistant cell line. Splicing modulation reverses aberrant BRAF splicing and slows growth of vemurafenib-resistant cells in vitro and in vivo using a xenograft model. Our results establish proof-of-principle for splicing modulation as a therapy for cancers with a molecular addiction to a weakly spliced oncogene isoform. Identification of an intronic BRAF vemurafenib resistance mutation To explore the molecular basis for the pre-mRNA splicing-mediated resistance to vemurafenib, we took advantage of the availability of vemurafenib-resistant C3 human melanoma cells [13] . These cells were generated by prolonged BRAF inhibitor treatment of SKMEL-239 cells, a patient-derived melanoma cell line expressing BRAF(V600E) [13] . Similar to the situation in vemurafenib-resistant patients, resistance in C3 cells is mediated by expression of the alternatively spliced BRAF3–9 isoform, which lacks exons 4–8 ( Fig. 1a ) [13] . Consistent with the heterozygous nature of the BRAF(V600E) mutation, we detected both BRAF3–9 and fully spliced BRAF (BRAF8–9) in the resistant C3 cells. No BRAF3–9 was detected in the parental cell line ( Fig. 1b and Supplementary Fig. 1a ). Elevated levels of BRAF3–9 in C3 cells were not due to nonsense-mediated degradation of other BRAF isoforms since silencing of UPF1, a component of the nonsense-mediated mRNA decay complex, did not affect BRAF3–9 or 7–9 isoforms ( Supplementary Fig. 1b, c ; P value <0.01). Comparative sequencing of genomic BRAF in C3 and their parental SKMEL-239 cells identified a C-to-G mutation at position 51nt upstream of the 3′ splice site (SS) of intron 8 in the BRAF(V600E) allele in C3 cells ( Supplementary Fig. 1d ). The −51 mutation maps to a predicted branch point (BP) in intron 8 (ref. 20 ). BRAF3–9 isoform formation by an intronic mutation The −51 BRAF mutation was sufficient to promote BRAF3–9 formation. In a BRAF minigene containing exons 3, 4, 8, 9 and parts of introns 3 and 8 ( Supplementary Fig. 1e ), the mutation favoured production of the BRAF3–9 isoform approximately two fold and reciprocally reduced BRAF8–9 as judged by quantitative PCR (qPCR) and semi-qPCR compared with the wild-type (wt) control ( Fig. 1c and Supplementary Fig. 1g ; P value<0.01). These effects were observed regardless of whether the reporters were introduced into parental or resistant C3 cells, excluding the possibility of cell-intrinsic effects on BRAF splicing ( Supplementary Fig. 1h ). In addition to the predicted intron 8 BP, sequence analysis [20] and secondary structure analysis [21] indicate the presence of two cryptic BPs (cBPs) located at positions −88 and −109 nt in intron 8, respectively, upstream of the 3′ SS ( Fig. 1d ). To test whether these cBPs are responsible for BRAF3–9 splicing in the presence of the −51 mutation in vemurafenib-resistant cells, we mutated the cBPs in the context of either wt or mutant BRAF ( Fig. 1e ). Mutation of both putative cBPs in the wtBRAF background only had a negligible effect on BRAF3–9 splicing ( Fig. 1e ). In contrast, mutation of these sites in the context of the −51 vemurafenib-resistant BRAF mutant resulted in a 40% decrease in BRAF3–9 usage ( Fig. 1e ; P value<0.05). In addition, mutation of a SRSF6-binding site at −129, but not of SRSF6 sites at exon 8, as well knockdown of SRSF6, but not SRSF1 or 3, in resistant C3 cells reduced endogenous BRAF3–9 by ∼ 30% ( Supplementary Fig. 1i and j ; P value<0.05) and in U2OS cells stably expressing the BRAF minigene ( Supplementary Fig. 1k and l ; P value<0.01). No differences in SRSF6 mRNA levels were found in parental and resistant cell lines before RNA interference (RNAi) treatment ( Supplementary Fig. 1m ). Splicing modulators reduce BRAF3–9 production and activity Given the shift in alternative splicing towards the BRAF3–9 isoform in vemurafenib-resistant cells, we tested whether treatment of resistant cells with the splicing modulator spliceostatin A (SSA) [22] or its analogue meayamycin B (MAMB) [23] , [24] , which target splicing factor SF3B1, inhibit BRAF3–9 formation. Treatment of C3-resistant cells with SSA (100 ng; 9 h) decreased the amount of BRAF3–9 in resistant C3 cells ( Fig. 2a ; P value<0.05). As a control, BRAF8–9 splicing was not affected by SSA treatment in either parental or resistant cell lines ( Fig. 2a and Supplementary Fig. 2a ). The effect of SSA was specific as ∼ 60% reduction of its immediate target SF3B1 by RNAi ( Supplementary Fig. 2b ; P value<0.01) mimicked these effects ( Supplementary Fig. 2c, d ; P value<0.05). Treatment with MAMB (10 nM; 9 h) had similar effects ( Fig. 2b ; Supplementary Fig. 2e ). As a further specificity control, we monitored the AS of the MAPK gene Erk-1 (ref. 25 ) and found no change in either parental or resistant cell lines ( Supplementary Fig. 2f ). As expected, reduction of BRAF3–9 splicing resulted in reduction of BRAF3–9 protein isoform in the resistant cell line ( Fig. 2c ) and was accompanied by a decrease in ERK signalling ( Fig. 2d and Supplementary Fig. 2g, h ; P value<0.05). As shown before [13] , total BRAF levels are lower in the resistant C3 cell line compared with parental ( Fig. 2c ), yet ERK activity is elevated in resistant cells ( Fig. 2d and Supplementary Fig. 2g, h ). We conclude that splicing interference antagonizes BRAF3–9 production. 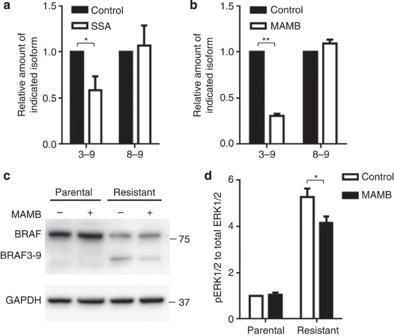Figure 2: Effect of splicing modulation on BRAF3–9 splicing. (a) Vemurafenib-resistant C3 cells were treated with 100 ng ml−1SSA for 9 h. mRNA levels were assessed using qPCR. Indicated isoform values are normalized to total BRAF mRNA. Isoform levels in the control were set to 1. (b) Vemurafenib-resistant C3 cells were treated with 10 nM MAMB for 9 h. mRNA levels were assessed using qPCR. Indicated isoform values are normalized to total BRAF mRNA. Isoform levels in the control were set to 1. (candd) Parental and resistant C3 cells were treated with 10 nM MAMB for 9 h. (c) Immunoblotting was conducted with the indicated antibodies, (d) BRAF activity was determined by measuring pERK1/2 levels using a Meso Scale Discovery (MSD) technology. For SSA, MAMB experiment control cells were treated with either methanol or dimethylsulphoxide, the compound solvent. (a,bandd) Values represent means of three independent experiments ±s.d. (*P<0.05, **P<0.01,t-test). GAPDH, glyceraldehyde 3-phosphate dehydrogenase. Figure 2: Effect of splicing modulation on BRAF3–9 splicing. ( a ) Vemurafenib-resistant C3 cells were treated with 100 ng ml −1 SSA for 9 h. mRNA levels were assessed using qPCR. Indicated isoform values are normalized to total BRAF mRNA. Isoform levels in the control were set to 1. ( b ) Vemurafenib-resistant C3 cells were treated with 10 nM MAMB for 9 h. mRNA levels were assessed using qPCR. Indicated isoform values are normalized to total BRAF mRNA. Isoform levels in the control were set to 1. ( c and d ) Parental and resistant C3 cells were treated with 10 nM MAMB for 9 h. ( c ) Immunoblotting was conducted with the indicated antibodies, ( d ) BRAF activity was determined by measuring pERK1/2 levels using a Meso Scale Discovery (MSD) technology. For SSA, MAMB experiment control cells were treated with either methanol or dimethylsulphoxide, the compound solvent. ( a , b and d ) Values represent means of three independent experiments ±s.d. (* P <0.05, ** P <0.01, t -test). GAPDH, glyceraldehyde 3-phosphate dehydrogenase. Full size image Splicing modulators inhibit vemurafenib-resistant cell proliferation As previously shown, vemurafenib-resistant C3 cells are dependent on BRAF3–9 for their proliferation [13] . To test whether splicing interference blocks proliferation of drug-resistant cells, we treated parental SKMEL-239 or resistant C3 cells for 3 days with MAMB. To ensure cell survival over 3 days of treatment, the dose range used (0.05–0.5 nM) was ∼ 50 times lower than the routine dose (10 nM) used for short-term splicing assays [26] . Resistant C3 cells were significantly more sensitive to MAMB compared with control parental cells in the absence of vemurafenib ( Fig. 3a ; P value<0.0001). The decreased proliferation rate in resistant C3 cells at a dose of 0.2 nM was accompanied by a reduction in the BRAF3–9 isoform ( Supplementary Fig. 3a, b ). Importantly, splicing interference re-sensitized resistant C3 cells to vemurafenib and reduced their proliferation potential to that of the drug-responsive parental cells ( Fig. 3b ; P value<0.001). Re-sensitization of C3 cells to vemurafenib was accompanied by a reduction of BRAF3–9 and consequently ERK signalling ( Supplementary Fig. 3c,d ; P value<0.05). Splicing modulation had no effect on proliferation, or ERK signalling, in the parental cell line ( Supplementary Fig. 3d, e ). These results demonstrate that SSA and MAMB reduce BRAF3–9 splicing and consequently ERK signalling. 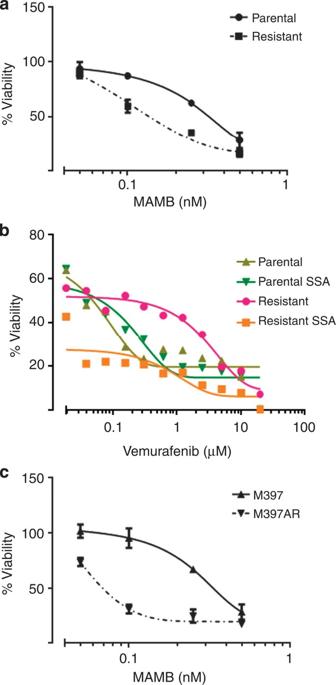Figure 3: Splicing modulation perturbs proliferation of resistant cell lines. (a) Parental and resistant C3 cells were treated with the indicated concentration of MAMB and cell viability was determined after 3 days. (b) Vemurafenib sensitivity curves at 3 days for parental and resistant C3 cells in the presence or absence of 1 ng ml−1of SSA. (c) Parental M397 and resistant M397AR cells were treated with the indicated concentration of MAMB and cell viability was determined after 3 days. Values represent means of three independent experiments±s.d. (P<0.001, two-way analysis of variance). Figure 3: Splicing modulation perturbs proliferation of resistant cell lines. ( a ) Parental and resistant C3 cells were treated with the indicated concentration of MAMB and cell viability was determined after 3 days. ( b ) Vemurafenib sensitivity curves at 3 days for parental and resistant C3 cells in the presence or absence of 1 ng ml −1 of SSA. ( c ) Parental M397 and resistant M397AR cells were treated with the indicated concentration of MAMB and cell viability was determined after 3 days. Values represent means of three independent experiments±s.d. ( P <0.001, two-way analysis of variance). Full size image An estimated 30% of vemurafenib-resistant tumours contain various BRAF splicing isoforms [13] , [19] ( Fig. 1a ). To test whether splicing interference is specific to BRAF3–9 or is also applicable to other BRAF isoforms, we treated the vemurafenib-resistant M397AR cell line, which expresses BRAF1–11, with MAMB (10 nM, 9 h) [12] , [27] . BRAF1–11 was reduced by 50% in the resistant M397AR cells ( Supplementary Fig. 3f ; P value<0.05). This effect was not due to general splicing suppression as BRAF10–11 splicing was only moderately decreased by MAMB treatment in either M397 or M397AR cell lines ( Supplementary Fig. 3f, g ). As observed for C3 cells, resistant M397AR cells were more sensitive to MAMB compared with control M397 cells ( Fig. 3c ; P value<0.0001). Furthermore, splicing modulation had no effect on proliferation in two sets of cell lines resistant to vemurafenib by non-RNA splicing-mediated mechanism [14] , [28] ( Supplementary Fig. 3h, i ). Splicing modulation inhibits growth of vemurafenib-resistant tumours in vivo To explore the potential use of splicing modulation in tumours in vivo , we performed xenograft experiments. Parental SKMEL-239 or vemurafenib-resistant C3 cells (1 × 10 6 ) were injected subcutaneously into immunocompromised NSG mice and animals were treated with a low dose of SSA (0.28 μg kg −1 ; injected ip every 3 days). Although SSA had no effect on tumour formation of parental cells, the formation of tumours by vemurafenib-resistant cells was effectively blocked in the presence of SSA ( Fig. 4a and Supplementary Fig. 4a ; P value<0.05). Vemurafenib-resistant tumours did not grow at all (3/4) or were at least ten times smaller in weight than the average parental tumour (1/4). To probe whether splicing modulation had any beneficial effect on already established vemurafenib-sensitive or -resistant tumours, NSG mice with clearly detectable 6-day-old SKMEL-239 or C3 tumours were treated with vemurafenib alone or in combination with SSA (0.28 μg kg −1 ; intraperitoneal (i.p.) injected every 3 days). As expected, vemurafenib reduced the size of SKMEL-293, but not of C3-tumours ( Fig. 4b ; Supplementary Fig. 4b ). SSA alone had no inhibitory effect and did not impede vemurafenib in drug-sensitive SKMEL-293 tumours ( Fig. 4b ). In contrast, SSA effectively inhibited tumour growth of vemurafenib-resistant C3 cells either alone or in combination with vemurafenib ( Fig. 4b and Supplementary Fig. 4c ; P value<0.05). Importantly, the reduction in tumour size observed in the resistant C3 tumours was accompanied by a decrease in BRAF3–9, but not BRAF8–9 ( Fig. 4c and Supplementary Fig. 4d ; P value<0.001). We conclude that elimination of the resistance-causing BRAF3–9 isoform by interference with pre-mRNA splicing is an effective means to overcome vemurafenib-resistance in-vivo . 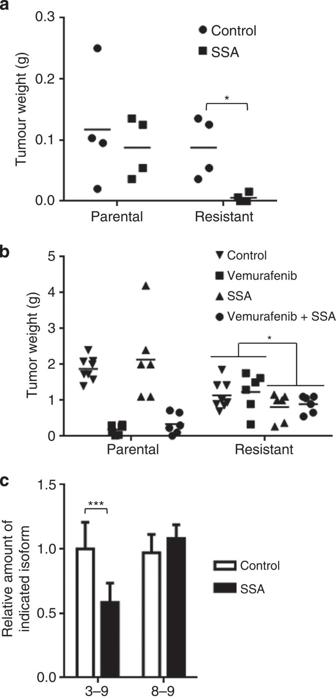Figure 4: SSA inhibits tumour growth of vemurafenib-resistant cells. (a) Values of tumour weight at the experiment end point (day 20) represent means±SEM from four mice (*P<0.05,t-test). (b) Tumours were formed for 6 days by injection of parental or resistant C3 cells and NSG mice then treated with vemurafenib analogue PLX4720 mixed in chow (417 mg drug per kg chow; 67 mg kg−1in mice) and/or 0.28 μg kg−1SSA. Values of tumour weight at the experiment endpoint (day 35) represent means±SEM from 6 mice (*P<0.05,t-test). (c) Quantitative PCR analysis of resistant C3 tumours with or without SSA. mRNA values are normalized to total BRAF mRNA. Control was set to 1. Values represent means of 6 mice ±s.d. (***P<0.001,t-test). Figure 4: SSA inhibits tumour growth of vemurafenib-resistant cells. ( a ) Values of tumour weight at the experiment end point (day 20) represent means±SEM from four mice (* P <0.05, t -test). ( b ) Tumours were formed for 6 days by injection of parental or resistant C3 cells and NSG mice then treated with vemurafenib analogue PLX4720 mixed in chow (417 mg drug per kg chow; 67 mg kg −1 in mice) and/or 0.28 μg kg −1 SSA. Values of tumour weight at the experiment endpoint (day 35) represent means±SEM from 6 mice (* P <0.05, t -test). ( c ) Quantitative PCR analysis of resistant C3 tumours with or without SSA. mRNA values are normalized to total BRAF mRNA. Control was set to 1. Values represent means of 6 mice ±s.d. (*** P <0.001, t -test). Full size image We identify here a point mutation in BRAF , which renders melanoma cells resistant to the clinically used BRAF inhibitor vemurafenib. The mutation is located in a putative splicing branch-point and promotes the generation of the BRAF3–9 splicing isoform, which confers vemurafenib resistance. We also find that several pre-mRNA splicing modulators, including SSA and MAMB, are able to counteract production of BRAF3–9 and overcome splicing-mediated vemurafenib resistance. The observed inhibitory effect of SSA on tumour formation of vemurafenib-resistant cells, even in the absence of the BRAF(V600E) inhibitor, indicates that elimination of the BRAF3–9 isoform is sufficient for a beneficial effect. This interpretation is in line with a dominant gain-of-function mechanism of BRAF3–9, which has constitutive BRAF activity due to loss of its RAS-binding domain (RBD) [13] . Although the prevalence of the −51 mutation is currently unknown, targeting of RNA splicing-mediated resistance to vemurafenib will possibly be of general clinical relevance as ∼ 30% of resistant tumours in patients treated with vemurafenib have been reported to express resistance-mediating BRAF splicing isoforms [9] , [13] , [19] . As all pre-mRNA splicing-mediated resistant tumours share common splicing isoforms that remove the RBD in BRAF [13] , it is anticipated that splicing interference may be effective regardless of the precise resistance mutation. This notion is supported by our finding that splicing interference also prevents production of the vemurafenib-resistant BRAF1–11 isoform. The dose of splicing modulators used in our experiments is significantly lower than that used in previous clinical trials of the SSA/MAMB analogue E7107-related (refs 29 , 30 ), reducing the risk of toxicity and suggesting its feasibility in a clinical setting. In support, low doses of SSA had no effect on growth of parental cells or tumours and showed no discernible toxicity in mice. Our results suggest that inhibition of splicing may be a complementary approach to currently used combination therapies of vemurafenib with MEK or histone deacetylases (HDAC) inhibitors [14] , [15] , [31] , [32] , [33] . Given the high prevalence of pre-mRNA splicing-mediated drug resistance, targeting pre-mRNA splicing may be a useful approach to overcome drug resistance in melanoma patients. Cell lines SKMEL-239 parental and vemurafenib-resistant C3 cell lines (a kind gift from David Solit, MSKC) as well as M397/M397AR (a kind gift from Antoni Ribas, UCLA), WM938B/WM983B BR and 451 Lu/451 Lu BR cell lines (a kind gift from Meenhard Herlyn, The Wistar Institute) were grown in RPMI supplemented with 10% fetal bovine serum. U2OS (ATCC Number: HTB-96) cells were grown in DMEM supplemented with 10% fetal bovine serum; all cell lines were maintained at 37 °C and 5% CO 2 atmosphere. Sequencing Sequencing was performed on purified PCR products of the 5′ SS of intron 3 and 3′ SS of intron 8 by GENEWIZ, Inc. BRAF reporter gene and transfection The reporter gene was constructed by stitching PCR products using GeneArt Seamless Cloning Technology (Life Technologies), and the product cloned into the pEGFP-N1 vector (Clontech). PCR reactions used to create wtBRAF and mutBRAF reporters were constructed using genomic DNA of parental or resistant C3 cell lines as template, respectively. Mutagenesis was performed using QuikChange II XL Site-Directed Mutagenesis Kit (Agilent Technologies). Cells were transfected using Nucleofector Technology (Lonza). Primers used in this study are provided in Supplementary Table 1 . RNAi OnTarget Plus SMARTpool against SF3B1, UPF1, SRSF1, SRSF3 and SRSF6 were obtained from Dharmacon (Lafayette). Cells were grown to 20–50% confluence and transfected with siRNA using the DharmaFECT 1 reagent (Lafayette). qPCR RNA was isolated from cells using the RNeasy plus mini kit (QIAGEN). cDNA synthesis was carried out with the High Capacity cDNA Reverse Transcription Kit (Applied Biosystems). qPCR was performed with the SsoFast EvaGreen Supermix (Bio-Rad) on the Biorad iCycler. The comparative Ct method was employed to quantify transcripts, and delta Ct was routinely measured in triplicate. Primers used in this study are provided in Supplementary Table 1 . Erk1 and cErk1 primers were designed elsewhere [25] . Secondary structure, BP and SRSF6-binding site prediction The full minigene sequence (2,684 nt) was folded using the Vienna RNAfold server ( http://rna.tbi.univie.ac.at/cgi-bin/RNAfold.cgi ) [21] to obtain the minimum free energy structure, the partition function and the base pairing probabilities. The results were cross-checked with the mfold server ( http://mfold.rna.albany.edu/?q=mfold ) [34] , [35] , [36] . The 3′ SS of intron 8 (1,000 nt) was analysed using ESEfinder 3.0 (ref. 20 ), to locate the BP and the two cBPs. The full minigene sequence (2,684 nt) was analysed using ESEfinder 3.0_ENREF_19 (ref. 20 to identify possible binding sites for SRSF6. Imaging Cells were fixed by adding 4% paraformaldehyde in PBS directly into the culture medium at a 1:1 para/medium ratio and incubated for 15 min at room temperature. Cells were then washed 3 × in PBS and stained with DRAQ5 (Biostatus Limited) 1:5,000 in PBS. Automated imaging steps were performed using an Opera system (Perkin-Elmer). Images were taken using a 488/640 nm excitation laser (first acquisition) and a 568 nm excitation laser (second acquisition). Images were analysed using the Acapella software package (Perkin-Elmer). The Green/Red ratio was calculated as the ratio between the average nuclear intensity signal in the 488-nm channel and the average nuclear signal in the 568-nm channel. Minimum of a 1,000 nuclei was analysed in each experiment condition. Transplantation assays Six-week-old male NOD/SCID/interleukin 2 receptor-γ null mice (NSG; Jackson Laboratory) were maintained in pathogen-free conditions. For generation of tumours, cells (1 × 10 6 per injection) in 35 μl of PBS were mixed with 15 μl of Matrigel (BD BioScience) and were injected subcutaneously into the flanks of mice. Mice were locally shaved with a depilatory cream 1 day before injection. SSA (0.28 μg kg −1 ) was injected i.p. (100 μl) every 3 days from the day indicated. Control mice were injected with PBS supplemented with methanol (SSA solvent). Vemurafenib analogue PLX4720 mixed in chow (417 mg drug per kg chow; 67 mg kg −1 in mice) was provided from day 6 for the duration of the experiment. Tumour growth was assessed twice a week using a digital caliper. Tumour volume was calculated according to the formula d × D , where d and D are the shortest and the longest diameter, respectively. At the end point, tumours were removed, weighted and RNA was extracted. All procedures were approved by the National Institutes of Health Animal Use and Care Committee. Proliferation assay Two thousand cells were seeded per well in a 96-well plate; the cells were treated the next day. SSA, MAMB or vemurafenib (PLX4032, Selleck) were mixed to the indicated dose. Control cells were treated with both dimethylsulphoxide and methanol or dimethylsulphoxide alone, the solvents of PLX4032, SSA and MAMB, respectively. Proliferation was assessed after 3 days by CellTiter 96 (Promega) according to the manufacture’s instructions. pERK1/2 assay Meso Scale Discovery plates were used for the detection of pERK1/2 and total ERK1/2, according to the manufacturer’s protocol. Plates were analysed on the SECTOR Imager. Immunoblotting Cells were harvested and lysed with RIPA lysis buffer supplemented with protease and phosphatase inhibitors, and the extracts were run on 4–12% Bis-Tris gel and transferred onto a polyvinylidene difluoride membrane. BRAF Antibody (F-7): sc-5284 (1:1,000), Anti-Hsc70 antibody [1B5] (ab19136, 1:25,000). How to cite this article : Salton, M. et al . Inhibition of vemurafenib-resistant melanoma by interference with pre-mRNA splicing. Nat. Commun. 6:7103 doi: 10.1038/ncomms8103 (2015).